Integrin CD11b negatively regulates BCR signalling to maintain autoreactive B cell tolerance A variant of the integrin-α-M ( CD11b ) gene has been linked to the pathogenesis of systemic lupus erythematosus. However, how this genotype results in the lupus phenotype is not fully understood. Here we show that autoreactive B cells lacking CD11b exhibit a hyperproliferative response to B cell receptor (BCR) crosslinking and enhanced survival. In vivo engagement of BCR in CD11b-deficient mice leads to increased autoAb production and kidney Ig deposition. In addition, CD11b-deficient autoreactive B cells have decreased tyrosine phosphorylation including Lyn and CD22 with decreased phosphatase SHP-1 recruitment but increased calcium influx. Results obtained using B cells transfected with the wild type or rs1143679 lupus-associated variant of CD11b suggest that this mutation completely abrogates the regulatory effect of CD11b on BCR signalling. This is through disruption of CD22–CD11b direct binding. These results reveal a previously unrecognized role of CD11b in maintaining autoreactive B cell tolerance. The hallmark of systemic lupus erythematosus (SLE) is the loss of immunological tolerance, and B cell hyperactivity. Autoantibodies (autoAbs) against macromolecular complexes, such as chromatin and small nuclear ribonucleoproteins (snRNPs), are predominant in SLE patients and have an important role in the pathogenesis of SLE [1] . The production of autoAbs is indicative of a profound breakdown of humoral tolerance mechanisms and B cell hyperactivity caused either by B cell intrinsic abnormalities or immunoregulatory defects of other cell types [2] . SLE predominantly affects women and has strong genetic component compared with many other autoimmune diseases. A number of candidate gene loci have been reported by genome-wide linkage studies in multiplex SLE families and by case–control studies [3] , [4] . A recent study reported an association between a variant at exon 3 (rs1143679) of integrin-α-M (CD11b, also called ITGAM , one subunit of complement receptor 3 (CR3)) and SLE susceptibility in individuals of European and African descent [5] . rs1143679 polymorphism converts the normal arginine at amino-acid position 77 to a histidine (R77H substitution). Subsequently, other groups independently reported an association between SLE susceptibility and intronic single nucleotide polymorphisms within ITGAM in populations of not only European ancestry but also in Hispanic- and African-Americans, Mexicans, Colombians, Hong Kong Chinese and Thai [5] , [6] , [7] , [8] , [9] . In addition, anti-double-stranded DNA autoAb production was associated in lupus patients with ITGAM gene variants [10] . Defect of a functional epitope of CR3 was also described in a SLE patient with immune vasculitis and panniculitis [11] . Collectively, these studies suggest that mutation within CD11b is a risk factor related to disease susceptibility, autoAb production and probably severe manifestations of SLE. CD11b, the 165-kDa ITGAM , non-covalently associates with CD18 to form α M β 2 , also known as macrophage-1 antigen (Ag) (Mac-1) or CR3. CR3/Mac-1 is a type I membrane glycoprotein and is one of four members of the leucocyte-restricted β 2 -integrin family [12] , [13] , [14] , [15] . Previous studies demonstrated that interaction of CD11b and complement component 3 (C3) activation product iC3b molecules is required for ultraviolet-induced immunosuppression and antigenic tolerance [16] . Ligation of CD11b by iC3b resulted in the production of anti-inflammatory cytokines such as interleukin-10 and transforming growth factor-β [17] . CD11b also facilitates oral tolerance by suppressing T-helper 17 cell differentiation [18] , negatively regulates natural killer cell activation and attenuates poly(I:C)-induced acute hepatitis [19] . Further, it was shown that CD11b negatively regulates Toll-like receptor-triggered inflammatory responses in macrophages [20] . However, the role of CD11b, particularly R77H mutation of CD11b in lupus disease pathogenesis has not been fully elucidated. In the present study, we find surprisingly that CD11b is critical in regulating B cell receptor (BCR)-mediated autoreactive B cell activation/tolerance. Autoreactive B cells from CD11b-knockout (KO) mice exhibit hyperproliferative responses on BCR crosslinking as a result of enhanced B cell proliferation and survival. This is specific for BCR signalling as other B cell stimuli including lipopolysaccharide (LPS) and CpG do not have such effect. In vivo BCR engagement by apoptotic cells further confirms that loss of CD11b results in the breakdown of autoreactive B cell tolerance. Our findings also indicate that CD11b negatively regulates BCR signalling through the Lyn–CD22–SHP-1 pathway. R77H mutation on CD11b completely abolishes this regulatory effect via the destruction of CD22–CD11b direct binding, suggesting that the non-functional CD11b (R77H) variant is associated with dysregulated B cell function. Thus, CD11b may serve as one of the threshold-setting molecules on B cells in the regulation of autoreactive B cell tolerance. CD11b is expressed on B cells in anti-snRNP Ig Tg mice CD11b is conventionally considered as a marker for myeloid cells. To investigate the CD11b expression patterns on B cells, we performed flow cytometric analyses of CD11b expression on different B cell populations from anti-snRNP immunoglobulin (Ig) transgenic (Tg) mice. As described previously, these B cells recognize autoAg Smith (Sm) [21] ; Sm is an ribonucleoprotein particle present in the nuclei of all cells and involves RNA processing [22] . Cells from the bone marrow (BM), spleen (Sp) and peritoneal cavity (Per) were stained with anti-B220 along with the following monoclonal Abs: CD43, anti-IgM, CD19, CD5 and CD11b. In the BM, Pro/pre B cells (fraction A–C) expressed relatively higher levels of CD11b as compared with pre B (fraction D), early B (fraction E) and mature B cells (fraction F; Fig. 1a ) [23] . In addition, CD11b was highly expressed on Sp marginal zone (MZ) B cells and Per B1 cells ( Fig. 1b,c ). Follicular (FO) B cells expressed low but detectable level of CD11b ( Fig. 1b ). This is also confirmed by western blot as well as reverse transcriptase–PCR analysis using highly purified FO B cells ( Supplementary Fig. S1a–d ). In addition, human peripheral B cells expressed considerable levels of CD11b ( Fig. 1d ). However, CD11b deficiency did not alter B cell development as evidenced by the normal BM cellularity ( Fig. 1a ) and splenic B cell numbers. Further, FO and MZ B cell numbers and Per B1-cell numbers were comparable ( Supplementary Fig. S1e ). These data suggest that CD11b is expressed on all stages and subsets of B cells in anti-snRNP Ig Tg mice at various levels. 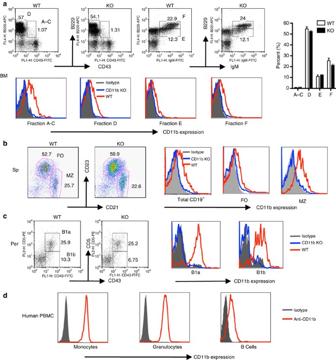Figure 1: CD11b expression on B cells in anti-snRNP Tg mice. (a) FACS analysis of BM lymphocytes stained with monoclonal Abs (mAbs) B220, CD43, IgM and CD11b. Comparison of B cell population within the BM lymphocyte gate is shown as means±s.e.m (n=4). (b) FACS analysis of splenocytes stained with mAbs CD19, CD21, CD23 and CD11b. Cells were gated on CD19+population. (c) FACS analysis of Per cells stained with mAbs B220, CD5, CD43 and CD11b. Cells were gated on B220+population. (d) FACS analysis of human peripheral blood cells stained with mAbs CD19 and CD11b. Cells were gated on monocytes, granulocytes and CD19+B cells. Results are representative of at least three independent experiments. Figure 1: CD11b expression on B cells in anti-snRNP Tg mice. ( a ) FACS analysis of BM lymphocytes stained with monoclonal Abs (mAbs) B220, CD43, IgM and CD11b. Comparison of B cell population within the BM lymphocyte gate is shown as means±s.e.m ( n =4). ( b ) FACS analysis of splenocytes stained with mAbs CD19, CD21, CD23 and CD11b. Cells were gated on CD19 + population. ( c ) FACS analysis of Per cells stained with mAbs B220, CD5, CD43 and CD11b. Cells were gated on B220 + population. ( d ) FACS analysis of human peripheral blood cells stained with mAbs CD19 and CD11b. Cells were gated on monocytes, granulocytes and CD19 + B cells. Results are representative of at least three independent experiments. Full size image CD11b KO B cells exhibit enhanced proliferation and survival To determine the effects of CD11b on anti-Sm B cells, splenic anti-Sm B cells from CD11b wild-type (WT) or KO B10.A anti-snRNP Ig Tg mice were stimulated with LPS, CpG or bivalent anti-IgM F(ab) 2 fragment (anti-IgM). B cell proliferation was measured by [ 3 H]-thymidine incorporation, direct cell counting and carboxyfluorescein succinimidyl ester dilution. As shown in Fig. 2a,b , anti-Sm B cells from CD11b KO mice exhibited hyperproliferation in response to anti-IgM stimulation. However, B cell proliferation on LPS or CpG stimulation was equivalent in both CD11b KO and WT Tg mice. This is particular for FO B cells but not for MZ B cells ( Supplementary Fig. S2a ). The hyperproliferation of anti-Sm B cells with CD11b deficiency was not the result of a change of surface IgM expression because the surface IgM level of CD11b KO anti-Sm B cells was comparable to that of WT B cells ( Supplementary Fig. S2b ), indicating that downstream signalling may be responsible for the hyperproliferation. 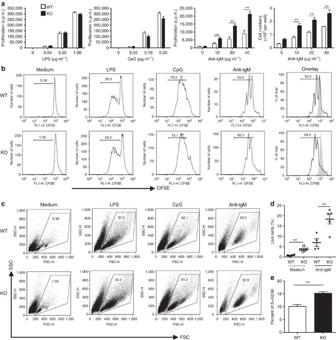Figure 2: CD11b-deficient B cells display enhanced responses to the BCR crosslinking but not Toll-like receptor ligands. (a) Purified B cells from CD11b KO and WT mice (n=5) were stimulated with LPS, CpG or anti-IgM for 48 h. B cell proliferation was assessed by [3H] thymidine incorporation. B cells stimulated with anti-IgM were also counted to obtain absolute number of live cells with trypan blue staining. (b) Carboxyfluorescein succinimidyl ester (CFSE)-labelled splenic B cells were incubated for 72 h in the presence or absence of LPS (0.1 μg ml−1), CpG (0.1 μg ml−1) or anti-IgM (40 μg ml−1). CFSE dilution was measured by flow cytometry. The overlaid histograms show proliferation of CD11b WT or KO B cells stimulated with anti-IgM compared with that of corresponding medium alone. (c) Purified B cells were stimulated with LPS, CpG or anti-IgM for 72 h. Viable cells were assessed by determining the FSC and SSC of cell populations by flow cytometry. (d) Purified B cells were cultured in medium or stimulated with anti-IgM for 72 h. Apoptotic cells were identified by staining with Annexin V and 7-AAD. Percentage of live cells is shown (n=5). Data are means±s.e.m. **P<0.01 (unpaired two-tailed Student’st-test). (e) Cell cycle analysis of B cells stimulated with anti-IgM for 48 h. The percentage of S phase and G2/M phase cells is shown (n=5). Data are means±s.e.m. **P<0.01 (unpaired two-tailed Student’st-test). Results are representative of at least three independent experiments. Figure 2: CD11b-deficient B cells display enhanced responses to the BCR crosslinking but not Toll-like receptor ligands. ( a ) Purified B cells from CD11b KO and WT mice ( n =5) were stimulated with LPS, CpG or anti-IgM for 48 h. B cell proliferation was assessed by [ 3 H] thymidine incorporation. B cells stimulated with anti-IgM were also counted to obtain absolute number of live cells with trypan blue staining. ( b ) Carboxyfluorescein succinimidyl ester (CFSE)-labelled splenic B cells were incubated for 72 h in the presence or absence of LPS (0.1 μg ml −1 ), CpG (0.1 μg ml −1 ) or anti-IgM (40 μg ml −1 ). CFSE dilution was measured by flow cytometry. The overlaid histograms show proliferation of CD11b WT or KO B cells stimulated with anti-IgM compared with that of corresponding medium alone. ( c ) Purified B cells were stimulated with LPS, CpG or anti-IgM for 72 h. Viable cells were assessed by determining the FSC and SSC of cell populations by flow cytometry. ( d ) Purified B cells were cultured in medium or stimulated with anti-IgM for 72 h. Apoptotic cells were identified by staining with Annexin V and 7-AAD. Percentage of live cells is shown ( n =5). Data are means±s.e.m. ** P <0.01 (unpaired two-tailed Student’s t -test). ( e ) Cell cycle analysis of B cells stimulated with anti-IgM for 48 h. The percentage of S phase and G2/M phase cells is shown ( n =5). Data are means±s.e.m. ** P <0.01 (unpaired two-tailed Student’s t -test). Results are representative of at least three independent experiments. Full size image Activated B cells upregulate co-stimulatory molecules (CD40, CD80 and CD86) and activation marker CD69. CD11b deficiency resulted in significantly upregulated expression levels of CD40, CD69, CD80 and CD86 on activated B cells ( Supplementary Fig. S2c ). We next sought to determine whether CD11b deficiency could enhance B cell survival or cell cycle progression. Purified B cells were stimulated with LPS, CpG or anti-IgM for 72 h. The viability of B cells was examined based on forward- and side-scatter characteristics. In accordance with the observed hyperproliferation of CD11b KO B cells, we recovered significantly more viable B cells from CD11b KO than WT B cells after anti-IgM stimulation. This phenomenon is specific for BCR stimulation, as CD11b KO B cells stimulated with LPS or CpG responded with similar changes ( Fig. 2c ). Further, B cell survival was quantified with Annexin V apoptosis detection kit. Significantly, more of CD11b KO B cells survived even without anti-IgM stimulation ( Fig. 2d ). Cell cycle analysis demonstrated that the entry into S and G2/M phases was significantly increased in CD11b KO B cells compared with that of WT B cells ( Fig. 2e ). In vivo 5-bromo-2-deoxyuridine (BrdU) incorporation assay revealed that CD11b KO B cells had significant lower turnover rate as compared with WT B cells ( Supplementary Fig. S2d ). Taken together, these data suggest that CD11b KO B cells proliferate more and die less as compared with WT B cells on BCR stimulation. We also found that messenger RNA expression levels of genes encoding anti-apoptotic proteins including stratifin (SFN) and STMN1 were markedly elevated in CD11b KO B cells ( Fig. 3a ). Western blot analysis revealed that protein expression levels of SFN and Bcl-xL were drastically increased even in the steady condition of B cells ( Fig. 3b and list of full blots). Thus, CD11b seems to maintain autoreactive B cell tolerance by negatively regulating B cell proliferation and survival. 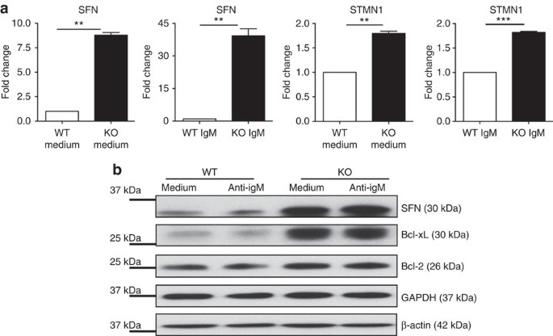Figure 3: CD11b-deficient B cells exhibit increased expression of anti-apoptotic genes and proteins. (a) Purified B cells were cultured in medium or stimulated with anti-IgM (40 μg ml−1) for 6 h. mRNA expression levels of SFN and STMN1 were measured using quantitative reverse transcriptase–PCR. Data are means±s.e.m. (n=3); **P<0.01; ***P<0.001 (unpaired two-tailed Student’st-test). (b) Purified B cells were stimulated with or without anti-IgM (40 μg ml−1) for 8 h and lysates were immunoblotted with SFN, Bcl-xL or Bcl-2 Abs. Results are representative of three independent experiments. Figure 3: CD11b-deficient B cells exhibit increased expression of anti-apoptotic genes and proteins. ( a ) Purified B cells were cultured in medium or stimulated with anti-IgM (40 μg ml −1 ) for 6 h. mRNA expression levels of SFN and STMN1 were measured using quantitative reverse transcriptase–PCR. Data are means±s.e.m. ( n =3); ** P <0.01; *** P <0.001 (unpaired two-tailed Student’s t -test). ( b ) Purified B cells were stimulated with or without anti-IgM (40 μg ml −1 ) for 8 h and lysates were immunoblotted with SFN, Bcl-xL or Bcl-2 Abs. Results are representative of three independent experiments. Full size image CD11b deficiency exaggerates autoAb responses in vivo Given that the CD11b deficiency led to enhanced B cell proliferation and survival in response to BCR stimulation in vitro , we investigated whether crosslinking of BCR in vivo would break autoreactive B cell tolerance to produce autoAb. Apoptotic cells are considered to be a major source for autoAgs in SLE [24] . AutoAgs associated with apoptotic blebs could efficiently stimulate B cells possibly by inducing multivalent crosslinking of BCR. Immunization of apoptotic cells resulted in the higher titre of anti-snRNP autoAb production in CD11b KO anti-snRNP Ig Tg mice as compared with that in WT mice ( Fig. 4a ). We also evaluated Ab-forming plasma cells (PCs) in these mice and found that CD11b KO mice had the higher frequency of CD19 + CD138 + PCs as compared with WT mice ( Fig. 4b ). In addition, the intensity of CD138 was also significantly higher in CD11b KO PC, suggesting the presence of a more activated anti-Sm CD138 high pre-PC subset, which occurs in murine SLE [25] . There were elevated serum levels of anti-nuclear antibodies (ANA; Fig. 4c ), and there was clear evidence of Ig deposition in kidney glomeruli in CD11b KO mice after immunization ( Fig. 4d ). 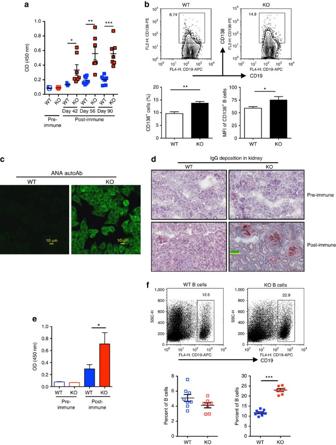Figure 4: CD11b-deficient mice develop enhanced snRNP autoAb response and kidney Ig deposition. (a) CD11b WT or KO B10.A anti-snRNP Tg mice (n=6 or 7) were immunized intravenously with apoptotic thymocytes weekly for 9 weeks. Sera were collected at indicated time points and anti-snRNP level was detected by ELISA. Data are means±s.e.m. (b) FACS analysis of CD138 expression on B cells from immunized mice (n=6 or 7). The percentage of CD138+cells (gated on CD19+population) and mean fluorescence intensity (MFI) of CD138+cells are shown. Data are means±s.e.m. (c) Serum ANA levels in immunized mice (scale bar, 10 μm). (d) Kidney sections from pre- or post-immunized WT or KO mice were probed with HRP-sheep anti-mouse IgG (1:25) to detect Ig deposition (dark red) in the glomeruli of immunized mice (scale bar, 50 μm). (e) Anti-snRNP level in sera of immunized Rag1-deficient mice (n=7 or 8) transferred with B cells from CD11b WT or KO anti-snRNP Ig Tg mice along with T cells (day 42). Data are means±s.e.m. (f) FACS analysis of CD19+cells in Sp from immunized Rag1-deficient mice (n=7 or 8). The percentages of B cells in peripheral blood from pre-immunized (left) and Sp in post-immunized (right) Rag1-deficient mice are shown. Data are means±s.e.m. *P<0.05; **P<0.01; ***P<0.001 (unpaired two-tailed Student’st-test). Figure 4: CD11b-deficient mice develop enhanced snRNP autoAb response and kidney Ig deposition. ( a ) CD11b WT or KO B10.A anti-snRNP Tg mice ( n =6 or 7) were immunized intravenously with apoptotic thymocytes weekly for 9 weeks. Sera were collected at indicated time points and anti-snRNP level was detected by ELISA. Data are means±s.e.m. ( b ) FACS analysis of CD138 expression on B cells from immunized mice ( n =6 or 7). The percentage of CD138 + cells (gated on CD19 + population) and mean fluorescence intensity (MFI) of CD138 + cells are shown. Data are means±s.e.m. ( c ) Serum ANA levels in immunized mice (scale bar, 10 μm). ( d ) Kidney sections from pre- or post-immunized WT or KO mice were probed with HRP-sheep anti-mouse IgG (1:25) to detect Ig deposition (dark red) in the glomeruli of immunized mice (scale bar, 50 μm). ( e ) Anti-snRNP level in sera of immunized Rag1-deficient mice ( n =7 or 8) transferred with B cells from CD11b WT or KO anti-snRNP Ig Tg mice along with T cells (day 42). Data are means±s.e.m. ( f ) FACS analysis of CD19 + cells in Sp from immunized Rag1-deficient mice ( n =7 or 8). The percentages of B cells in peripheral blood from pre-immunized (left) and Sp in post-immunized (right) Rag1-deficient mice are shown. Data are means±s.e.m. * P <0.05; ** P <0.01; *** P <0.001 (unpaired two-tailed Student’s t -test). Full size image It is noteworthy that studies shown above utilized CD11b global KO mice. B cell development and maturation require growth factors such as interleukin-7. To determine whether CD11b expression on the BM microenvironment has impact on autoreactive B cell tolerance, we established BM chimeras. Recipient WT or CD11b KO anti-snRNP Ig Tg mice were lethally irradiated with 950 cGy. BM cells from WT or CD11b KO Tg mice were adoptively transferred into recipient mice. Recipient mice were reconstituted with donor cells around 28 days after irradiation. Enhanced B cell proliferation ( Supplementary Fig. S3a ) and survival ( Supplementary Fig. S3b ) on BCR crosslinking occurred in KO–KO BM chimeric mice as compared with these in WT–WT BM chimeric mice. Similarly, enhanced B cell proliferation ( Supplementary Fig. S3a ) and survival ( Supplementary Fig. S3b ) on BCR crosslinking were observed in KO–WT BM chimeric mice as compared with those in WT–KO BM chimeric mice, suggesting that CD11b on the BM microenvironment does not influence regulatory effect of CD11b on autoreactive B cell activation/tolerance. To further rule out the possibility that altered B cell function is due to defective CD11b regulation on other cells, we used Rag1-deficient mice that were adoptively transferred with WT or KO B cells along with T cells. These mice were then immunized with apoptotic cells. Mice adoptively transferred with KO B cells produced significantly more autoAbs than mice transferred with WT B cells ( Fig. 4e ). These mice also had more CD19 + CD138 + PC and sera contained ANA autoAb ( Supplementary Fig. S3c ). Strikingly, B cells were significantly more in mice transferred with KO B cells as compared with mice transferred with WT B cells ( Fig. 4f ), suggesting survival advantage for KO B cells. We also used B cell-deficient μMT mice that were adoptively transferred with WT or KO B cells only. Consistent with previous findings in Rag1-deficinet mice, μMT mice transferred with KO B cells produced significantly more autoAbs than those transferred with WT B cells ( Supplementary Fig. S3d ), suggesting an intrinsic defect of CD11b KO B cells. Impaired Lyn–CD22–SHP-1-negative circuit in CD11b KO B cells A feature of BCR signalling is that it results in the phosphorylation of a wide array of signalling components [2] . Thus, we assessed the influence of CD11b deficiency on the level of protein tyrosine phosphorylation. Immunoblotting of anti-IgM-stimulated B cells revealed an altered protein tyrosine phosphorylation pattern in CD11b KO anti-Sm B cells compared with WT controls ( Fig. 5a ). Some unidentified tyrosine-phosphorylated protein bands were significantly decreased in CD11b KO B cell lysates ( Fig. 5a arrows). Although phosphorylated Sp tyrosine kinase (Syk), AKT, p38 MAPK and Erk1/2 were not significantly altered ( Fig. 5b and list of full blots), CD11b KO B cells exhibited decreased Lyn phosphorylation ( Fig. 5c and list of full blots). CD22 is an important molecule to inhibit BCR signalling [26] . CD22 can be quickly phosphorylated by Lyn after BCR crosslinking, thus generating docking sites for different signalling molecules. Phosphatases including the SH2-containing inositol 5-phosphatase (SHIP-1) and the SH2-containing phosphotyrosine phosphatase (SHP-1) can be recruited to the BCR/CD22 complex, thus negatively regulating BCR signalling [27] , [28] . However, the total protein levels of CD22, SHP-1 and SHIP-1 were not altered in CD11b KO B cells ( Fig. 5d and list of full blots). Next, we immunoprecipitated CD22 and found that phospho-CD22 level was drastically decreased in CD11b KO B cells on BCR crosslinking ( Fig. 5e and list of full blots). Subsequently, SHP-1 recruitment was also decreased. This was consistent with lower levels of Lyn expression associated with CD22 in CD11b KO B cells ( Fig. 5e ). 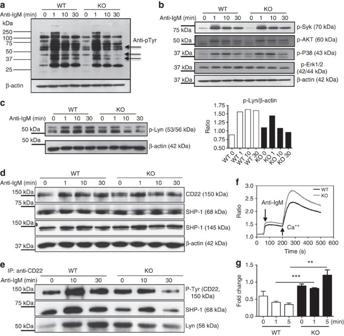Figure 5: BCR crosslinking induces decreased tyrosine phosphorylation and decreased recruitment of SHP-1 in CD11b-deficient B cells. (a–d) Purified B cells were stimulated with or without anti-IgM (40 μg ml−1) at indicated time points. Cell lysates were separated by SDS–polyacrylamide gel electrophoresis and blotted for total protein tyrosine phosphorylation (a), phospho-Syk, phospho-AKT, phospho-p38 and phospho-Erk1/2 (b), phospho-Lyn (c), CD22, SHP-1 and SHIP-1 (d). Relative amounts of phospho-Lyn were quantified with ImageJ software. (e) Lysates from WT and KO B cells were immunoprecipitated with anti-CD22 and protein A/G agarose. Tyrosine phosphorylation of CD22 was visualized by blotting with phosphotyrosine Ab. The membrane was stripped and reblotted with SHP-1 and Lyn Abs. (f) Calcium flux was monitored in Indo-1-loaded B cells stimulated with anti-IgM (40 μg ml−1). Arrows indicate the time points when anti-IgM or CaCl2was added. (g) The gene expression of STIM-1 was measured using quantitative reverse transcriptase–PCR (n=4). Data are means±s.e.m. **P<0.01; ***P<0.001 (unpaired two-tailed Student’st-test). Results are representative of three independent experiments. Figure 5: BCR crosslinking induces decreased tyrosine phosphorylation and decreased recruitment of SHP-1 in CD11b-deficient B cells. ( a – d ) Purified B cells were stimulated with or without anti-IgM (40 μg ml −1 ) at indicated time points. Cell lysates were separated by SDS–polyacrylamide gel electrophoresis and blotted for total protein tyrosine phosphorylation ( a ), phospho-Syk, phospho-AKT, phospho-p38 and phospho-Erk1/2 ( b ), phospho-Lyn ( c ), CD22, SHP-1 and SHIP-1 ( d ). Relative amounts of phospho-Lyn were quantified with ImageJ software. ( e ) Lysates from WT and KO B cells were immunoprecipitated with anti-CD22 and protein A/G agarose. Tyrosine phosphorylation of CD22 was visualized by blotting with phosphotyrosine Ab. The membrane was stripped and reblotted with SHP-1 and Lyn Abs. ( f ) Calcium flux was monitored in Indo-1-loaded B cells stimulated with anti-IgM (40 μg ml −1 ). Arrows indicate the time points when anti-IgM or CaCl 2 was added. ( g ) The gene expression of STIM-1 was measured using quantitative reverse transcriptase–PCR ( n =4). Data are means±s.e.m. ** P <0.01; *** P <0.001 (unpaired two-tailed Student’s t -test). Results are representative of three independent experiments. Full size image Calcium flux after BCR crosslinking is a central component of BCR signalling and is negatively regulated by CD22 (ref. 29 ). We found that B cells from CD11b KO B cells had increased calcium flux on BCR crosslinking as compared with WT B cells ( Fig. 5f ). This is also associated with rapidly increased mRNA levels of calcium sensor protein STIM-1 ( Fig. 5g ). Taken together, these data suggest that CD11b is essential to form BCR-induced Lyn-, CD22- and SHP-1-negative circuit. CD11b variant abolishes its regulatory effect on BCR signalling SLE has been found to be associated with a single nucleotide polymorphism rs1143679 located in the CD11b β-propeller domain [5] , which results in an arginine-to-histidine substitution at position 77 (R77H). To examine the effect of human WT and R77H-mutated CD11b on B cells, we used the mouse B cell line K46-17 μmλ (K46-17) that does not express CD11b to generate stable transfectants with equivalent expression of either WT human CD11b or R77H CD11b (CD11b Mut; Supplementary Fig. S4 ). Mouse CD11b is highly similar to its human counterpart with an overall sequence identity of 81% (ref. 30 ). Indeed, human CD11b can be paired with mouse CD18 to form surface-expressing CR3 ( Supplementary Fig. S4c ). K46-17 expresses surface IgM but not CD11b and exhibits a calcium response characterized by a biphasic phenotype [31] . WT CD11b expression significantly decreased calcium influx on BCR crosslinking ( Fig. 6a ). Strikingly, R77H mutation on CD11b molecule completely abolished WT CD11b-mediated downregulation of calcium influx ( Fig. 6b ). The level of calcium influx in K46-17/CD11b Mut was similar as that in K46-17 cells transfected with control vector. 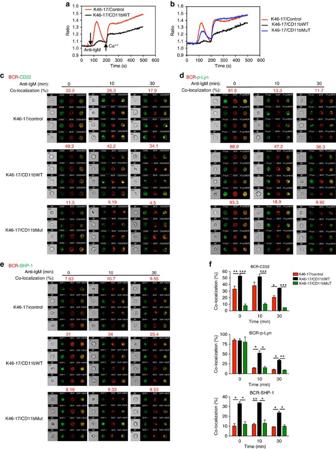Figure 6: R77H mutation abrogates CD11b inhibitory function on BCR signalling. (a,b) Calcium flux was monitored in CD11b WT- and CD11b Mut-expressing B cell lines stimulated with anti-IgM (5 μg ml−1). Control vector-transfected cells were also used. (c–e) Representative images showing co-localizations of BCR–CD22, BCR–p-Lyn and BCR–SHP-1. CD11b WT- or R77H mut-transfected B cell lines were stimulated with or without anti-IgM (5 μg ml−1) at indicated time points and stained with Abs against BCR, CD22, SHP-1 and phospho-Lyn. Percentage indicates cells demonstrating co-localizations of two molecules with similarity score >2. (f) Percentages of co-localized cells were summarized (n=2). Data are shown as means±s.e.m. *P<0.05; **P<0.01; ***P<0.001 (unpaired two-tailed Student’st-test). Results are representative of two independent experiments. Figure 6: R77H mutation abrogates CD11b inhibitory function on BCR signalling. ( a , b ) Calcium flux was monitored in CD11b WT- and CD11b Mut-expressing B cell lines stimulated with anti-IgM (5 μg ml −1 ). Control vector-transfected cells were also used. ( c – e ) Representative images showing co-localizations of BCR–CD22, BCR–p-Lyn and BCR–SHP-1. CD11b WT- or R77H mut-transfected B cell lines were stimulated with or without anti-IgM (5 μg ml −1 ) at indicated time points and stained with Abs against BCR, CD22, SHP-1 and phospho-Lyn. Percentage indicates cells demonstrating co-localizations of two molecules with similarity score >2. ( f ) Percentages of co-localized cells were summarized ( n =2). Data are shown as means±s.e.m. * P <0.05; ** P <0.01; *** P <0.001 (unpaired two-tailed Student’s t -test). Results are representative of two independent experiments. Full size image We next utilized these three B cell lines to delineate how WT or R77H-mutated CD11b has an impact on phospho-Lyn-, CD22- and SHP-1-negative circuit. The data were analysed using ImageStream. Percent of co-localization was determined by the similarity score greater than 2 ( Supplementary Fig. S5a,b ). Non-stimulated B cells with WT CD11b demonstrated more BCR–CD22 and BCR–SHP-1 co-localizations ( Fig. 6c–f ). CD11b Mut significantly decreased co-localizations of BCR–CD22 and BCR–SHP-1 but not BCR–p-Lyn co-localization, similar to B cells without CD11b expression (K46-17/control). BCR ligation resulted in minor dissociation of CD22 and SHP-1 from BCR and brisk dissociation of p-Lyn from BCR in K46-17/CD11b WT B cells. In contrast, significantly more dissociation of p-Lyn from BCR was observed in K46-17/CD11b Mut B cells. In these cells, CD22, p-Lyn and SHP-1 re-localized from BCR to opposite poles of the cell, similar to K46-17 B cells without CD11b expression. The differential localization of p-Lyn, CD22 and SHP-1 with BCR in B cells with WT CD11b versus B cells with CD11b Mut is further consistent with the regulation of BCR signalling by CD11b via Lyn–CD22–SHP-1-negative circuit. R77H mutation abrogates CD11b–CD22 direct binding To determine direct interaction among CD11b, CD22, p-Lyn, SHP-1 and BCR, B cells transfected with WT CD11b or R77H CD11b Mut were stimulated with or without BCR ligation. WT CD11b showed significant co-localizations with CD22, p-Lyn, SHP-1 and BCR ( Fig. 7a–e ). BCR ligation led to dramatic dissociation of CD11b–BCR complex and this was not significantly influenced by R77H mutation ( Fig. 7d ). Co-localizations of CD11b with CD22, p-Lyn and SHP-1 were not significantly altered on BCR ligation. However, R77H mutation significantly decreased co-localizations of these molecules ( Fig. 7a–c ). We further immunoprecipitated CD22 from CD11b WT- or R77H Mut-expressing B cells and found that Flag signal (CD11b) was significantly decreased in CD11b Mut B cells ( Fig. 7f and list of full blots), suggesting direct association between CD11b and CD22 molecules and R77H mutation disrupts CD11b-mediated negative regulation via the Lyn–CD22–SHP-1 pathway. 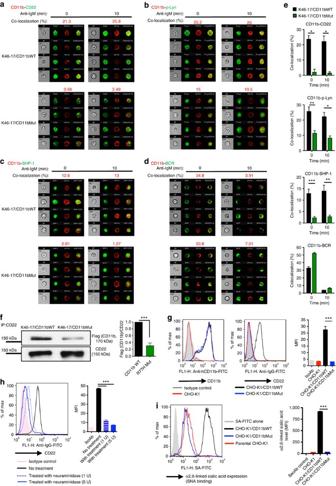Figure 7: CD11b R77H mut significantly reduces the co-localizations of CD11b with the components of Lyn-CD22-SHP-1-negative circuit and abolishes direct binding with CD22. (a–d) Representative images and percentages of cells showing co-localizations of CD11b–CD22, CD11b–p-Lyn, CD11b–SHP-1 and CD11b–BCR with similarity score >2. (e) Percentages of co-localized cells were summarized. (f) Immunoblotting for Flag (CD11b) and CD22 after CD22 immunoprecipitation from CD11b-transfected B cell lines. Relative amounts of Flag (CD11b) were quantified with ImageJ software. (g) Left panel, CD11b expression on stably transfected CHO-K1 cells; middle panel, CHO-K1 cells transfected with WT or R77H mut CD11b were incubated with recombinant human CD22 his tag protein. Binding of CD22 was probed with mouse his tag monoclonal Ab followed with anti-mouse IgG-FITC and was analysed by flow cytometry. Right panel, MFI of CD22 binding to CD11b-transfected CHO-K1 cells was summarized. (h) CD11bWT-transfected CHO-K1 cells were pretreated with neuraminidase (1U or 5U) and then were incubated with recombinant human CD22 his tag protein. (i) CD11b WT- or R77H CD11b-transfected CHO-K1 cells were stained with biotinylated lectinS. nigrafor 60 min and then stained with SA-FITC. The expression levels of α2,6-linked sialic acids were detected by flow cytometry and quantified by MFI. Data are shown as means±s.e.m. *P<0.05; **P<0.01; ***P<0.001 (unpaired two-tailed Student’st-test). Results are representative of two independent experiments for all panels. Figure 7: CD11b R77H mut significantly reduces the co-localizations of CD11b with the components of Lyn-CD22-SHP-1-negative circuit and abolishes direct binding with CD22. ( a – d ) Representative images and percentages of cells showing co-localizations of CD11b–CD22, CD11b–p-Lyn, CD11b–SHP-1 and CD11b–BCR with similarity score >2. ( e ) Percentages of co-localized cells were summarized. ( f ) Immunoblotting for Flag (CD11b) and CD22 after CD22 immunoprecipitation from CD11b-transfected B cell lines. Relative amounts of Flag (CD11b) were quantified with ImageJ software. ( g ) Left panel, CD11b expression on stably transfected CHO-K1 cells; middle panel, CHO-K1 cells transfected with WT or R77H mut CD11b were incubated with recombinant human CD22 his tag protein. Binding of CD22 was probed with mouse his tag monoclonal Ab followed with anti-mouse IgG-FITC and was analysed by flow cytometry. Right panel, MFI of CD22 binding to CD11b-transfected CHO-K1 cells was summarized. ( h ) CD11bWT-transfected CHO-K1 cells were pretreated with neuraminidase (1U or 5U) and then were incubated with recombinant human CD22 his tag protein. ( i ) CD11b WT- or R77H CD11b-transfected CHO-K1 cells were stained with biotinylated lectin S. nigra for 60 min and then stained with SA-FITC. The expression levels of α2,6-linked sialic acids were detected by flow cytometry and quantified by MFI. Data are shown as means±s.e.m. * P <0.05; ** P <0.01; *** P <0.001 (unpaired two-tailed Student’s t -test). Results are representative of two independent experiments for all panels. Full size image As CD22 is a B cell surface lectin receptor and can recognize α2,6-linked sialic acid containing glycoconjugates and negatively regulates BCR signalling [32] , we reasoned whether WT CD11b could serve as an endogenous ligand for CD22 binding. To this end, WT or R77H-mutated human CD11b was transfected into mammalian cell line CHO-K1 cells. Both cells expressed comparable levels of CD11b ( Fig. 7g ). Strikingly, CD22 only bound to WT CD11b but not to mutated CD11b ( Fig. 7g ). In addition, WT CD11b treated with neuraminidase had significantly decreased CD22 binding ( Fig. 7h ). We also directly measured the expression levels of α2,6-linked sialic acids using Sambucus nigra lectin-binding assay [33] . WT CD11b-transfected CHO-K1 cells, but not R77H-transfected or parental CHO-K1 cells exhibited profoundly lectin binding ( Fig. 7i ), suggesting that R77H mutation alters CD11b glycosylation leading to the loss of CD22-binding ability. In this study, we show a novel role of integrin CD11b in the maintenance of autoreactive B cell tolerance by providing negative regulation on BCR-mediated signalling via the Lyn–CD22–SHP-1 pathway. Historically, splenic B2 cells are not thought to express CD11b. However, a recent study showed that expression of CD11b on B cell is regulated via a negative feedback loop by the environment. Splenic B cells from C3-deficient mice have increased CD11b expression, whereas the presence of the ligand for CR3 decreases cell surface expression and transcripts of the CD11b [34] . In human, most CD27 + memory cells are CD11b positive [35] . Here we show that CD11b is constitutively expressed on all B cell subsets in anti-snRNP Tg mice, with various expression levels. Loss of CD11b on B cells leads to strikingly enhanced autoreactive B cell activation, differentiation and survival on BCR crosslinking. This is shown in both in vitro studies and in vivo BCR ligation. Recent studies also suggest that R77H mutation compromises CR3 effector functions including leucocyte adhesion and phagocytosis in human myeloid cells [36] , [37] , [38] . However, elevated autoAb production and B cell activation are mainly due to CD11b deficiency on B cells. This is demonstrated in BM chimeric mice and Rag1-deficient mice or B cell-deficient μMT mice transferred with WT or KO B cells. The increased autoreactive B cell survival in CD11b KO B cells is possibly caused by the activation of anti-apoptotic pathways including SFN pathway. It is interesting that a recent study demonstrated a critical role of SFN in regulating B cell homoeostasis [39] . Loss of SFN results in the increased B cell apoptosis. This is consistent with our finding that CD11b KO autoreactive B cells have higher mRNA and protein expression levels of SFN and Bcl-xL even in the steady condition as compared with WT B cells. BCR stimulation in CD11b KO mice induces the increase of SFN and STMN1 mRNA levels, indicating that CD11b signalling provides a negative feedback on autoreactive B cell survival. BCR signalling has critical roles in regulating B cell activation and anergy [40] . As apoptotic cells are constantly present in the circulation as a result of programmed cell death, autoreactive B cells encountering these apoptotic cells may be in the risk of subsequent activation. Thus, maintaining peripheral tolerance of autoreactive B cells is necessary to ensure unwanted, pathogenic autoimmune responses. Our data suggest that CD11b on B cells may have such role. Consequently, deficiency of CD11b on autoreactive B cells leads to enhanced proliferation and activation. Crosslinking of the BCR is rapidly followed by the recruitment of cytosolic protein tyrosine kinases [41] . Phosphorylation of the BCR components results in the recruitment and activation of Syk, which is essential for propagating BCR signalling [41] , [42] and is involved in the initiation of a series of mechanisms for negative regulation. For example, the kinase Lyn functions to phosphorylate immunoreceptor tyrosine-based activation motifs on inhibitory receptors such as CD22 to facilitate the recruitment of negative regulators of BCR signalling, including phosphatases SHP-1 and SHIP-1 (refs 28 , 43 ). Mice lacking Lyn or expressing constitutively active Lyn develop circulating autoAbs and severe autoimmune glomerulonephritis [44] . CD11b KO B cells display significantly decreased Lyn activity and subsequent decreased CD22 phosphorylation and SHP-1 recruitment, suggesting a critical role of CD11b in establishing the Lyn–CD22–SHP-1-negative circuit that is essential for the maintenance of autoreactive B cell tolerance [45] . How does CD11b molecule regulate the Lyn–CD22–SHP-1-negative circuit? We found that CD11b co-localizes with BCR and CD22 to form BCR–CD11b–CD22 receptor complex on B cell surface. In the steady condition, BCR and CD11b co-localize with p-Lyn and SHP-1, respectively, to ensure autoreactive B cell quiescence. On BCR ligation, BCR is quickly dissociated from CD11b molecule. However, co-localizations of BCR–CD22, BCR–SHP-1, CD11b–CD22, CD11b–p-Lyn and CD11b–SHP-1 are not significantly altered, suggesting that CD11b binding to CD22 stabilizes phospho-Lyn and CD22 and subsequent SHP-1 recruitment. This may be critical to set a threshold for autoreactive B cell activation while positive regulators for BCR signalling such as Syk are not altered by CD11b deficiency. Thus, the net outcome of autoreactive B cells on BCR ligation in the absence of CD11b is tilted towards enhanced proliferation and activation. This is consistent with decreased calcium influx level when WT CD11b is expressed on B cells. Strikingly, R77H mutation on CD11b significantly decreases co-localizations of BCR–CD22, BCR–p-Lyn and BCR–SHP-1 on BCR crosslinking. Although R77H mutation does not influence CD11b–BCR co-localization, co-localizations of CD11b with CD22, p-Lyn and SHP-1 are drastically decreased. These findings suggest that the R77 position on CD11b is essential to form CD11b–CD22 receptor complex on B cell surface. Consequently, augmented calcium influx is observed in B cells transfected with CD11b Mut. Thus, CD22 seems to be essential for CD11b-mediated negative regulation on BCR signalling. CD22 is a 140-kDa glycoprotein on the B cell surface and can be activated in trans on adjacent cells or cis on the same cell surface by different ligands including soluble IgM, CD45 and CD22 itself [46] , [47] . Clearly, WT CD11b can directly interact with CD22. This is demonstrated by the pull-down experiment and direct binding assay. This interaction is critical for CD22 activation and subsequent SHP-1 recruitment to form a negative regulatory circuit for BCR signalling. In contrast, R77H mutation significantly diminishes physical interaction between these two molecules. Our data further suggest that R77H mutation alters CD11b glycosylation because the expression of α2,6-linked sialic acid is completely lost on R77H-transfected cells. Consequently, R77H-mutated CD11b lose its binding ability to CD22 resulting in the impaired negative regulatory function of WT CD11b on B cells, leading to breakdown of autoreactive B cell tolerance. Future studies will be necessary to understand precisely how CD11b regulates human autoreactive B cells in lupus patients and to develop novel compounds to circumvent the defective regulatory role of CD11b mutations. Mice B10.A or C57Bl/6 anti-snRNP Ig Tg mice were described previously [48] and were crossed with CD11b KO mice (Jackson Laboratory) to generate CD11b KO anti-snRNP Ig Tg mice. These mice have been backcrossed onto B10.A or C57Bl/6 background for more than nine generations. B6. Rag1 -deficient mice (B6.129S7- Rag1 tm1Mom /J) and B6 μMT mice (B6.129S2- Igh-6 tm1Cgn /J) were obtained from Jackson Laboratory. Mice at 6–8 weeks of age with both sexes were used for experiments. All mice were housed and bred in a conventional facility at the University of Louisville. Animal care and experiments were conducted in accordance with the National Institutes of Health guidelines and were approved by the Institutional Animal Care and Use Committee at the University of Louisville. Reagents and cell line Fluorochrome-labelled Abs against mouse CD43 (S11, 1:100), CD45R/B220 (RA3-6B2, 1:500), IgM (RMM-1, 1:100), CD11b (M1/70, 1:500), CD19 (6D5, 1:500), CD21 (7G6, 1:100), CD23 (B3B4, 1:500), CD5 (53-7.3, 1:500), CD138 (281-2, 1:200), Gr-1 (RB6-8C5, 1:200), F4/80 (BM8, 1:200), NK1.1 (PK136, 1:200), anti-mouse IgG (1:100) and anti-human CD11b (ICRF44, 1:20) were purchased from BioLegend (San Diego, CA). Anti-BrdU (BU20A, 1:100) was purchased from eBioscience (San Diego, CA). Anti-his (HIS-1, 1:100) was from Sigma-Aldrich (St Louis, MO). Polyclonal CD11b (1:600), SFN (1:500) and Lyn (phospho Y396, 1:100) Abs were from Abcam (Cambridge, MA). Abs against Bcl-xL (1:1000), Bcl-2 (1:1000), phospho-Syk (Tyr352, 1:1000), phospho-Akt (Ser473, 1:1000), phospho-p38 MAPK (Thr180/Tyr182, 1:1000), phospho-Erk1/2 (Thr202/Tyr204, 1:1000), Lyn (1:1000), SHP-1 (1:1000), SHIP-1 (1:1000) and Flag (1:1000) were obtained from Cell Signaling Technology Inc. (Beverly, MA). Anti-phospho-Lyn (Tyr507, 1:2000) and anti-phosphotyrosine (4G10, 1:1000) was from EMD Millipore (Billerica, MA). Anti-rat IgG-HRP (1:5000) was from Santa Cruz Biotechnology, and anti-mouse IgG-HRP (1:3000) and anti-rabbit IgG-HRP (1:3000) were from GE Healthcare. Recombinant human CD22 protein (His tag) was purchased from Life Technologies (Grand Island, NY). The plasmid for human CD11b (plasmid 8631) and control plasmid c-Flag pcDNA3 (plasmid 20011) were obtained from Addgene (Cambridge, MA). The B-lymphoma cell line K46-17 μmλ (K46-17) was generously provided by Dr. John C. Cambier. Flow cytometry Single-cell suspensions were blocked in the presence of anti-CD16/CD32 at 4 °C for 15 min and stained on ice with the appropriate antibodies and isotype controls in PBS buffer containing 1% fetal bovine serum. The samples were acquired using FACSCalibur cytometer (BD Bioscience, San Jose, CA) and analysed using FlowJo software (Tree Star, Ashland, OR). In vitro B cell analysis and survival assay Splenic B cells were purified by negative selection by using anti-mouse CD43 microbeads and autoMACS (Miltenyi Biotech, Auburn, CA), as described previously [21] . In brief, splenocytes were incubated with anti-mouse CD43 microbeads for 30 min on ice. Cells were washed three times and then applied on autoMACS using negative selection mode. The purity of B cells was >95% as assessed by flow cytometry. In some experiments, splenocytes were stained with anti-CD19, anti-CD21 and anti-CD23. Total B cells (CD19 + ), FO B cells (CD19 + CD23 high CD21 low ) and MZ B cells (CD19 + CD23 − CD21 + ) were highly purified using FACSAria III cell sorter to a purity in excess of 99.5%. B cell proliferation was performed in RPMI 1640 medium (Caisson Laboratories, Logan, UT), supplemented with 10% inactivated fetal bovine serum, 10 –3 M sodium pyruvate, 2 × 10 –3 M glutamine and 50 μM 2-mercaptoethanol. B cells (1 × 10 5 per well, 96-well plate) were stimulated with varying amounts of LPS, CpG or anti-mouse IgM F(ab′) 2 (Jackson ImmunoResearch Laboratories, West Grove, PA) and proliferation was determined by [ 3 H]-TdR incorporation after 48 h of culture. Absolute numbers of live cells were also counted with trypan blue staining. Experiments were conducted in triplicate and results were expressed as c.p.m.±s.e.m. In some experiments, B cells were labelled with carboxyfluorescein diacetate succinimidyl ester (Life Technologies) before stimulation and analysed 3 days later. For cell cycle analysis, purified B cells were stimulated for 48 h with 40 μg ml −1 of anti-IgM. Subsequently, the cells were fixed with cold ethanol (70%) and treated with RNase. The nuclear DNA was labelled with propidium iodide and analysed by flow cytometry. For cell survival assay, B cells were cultured in medium alone or were stimulated with 40 μg ml −1 of anti-IgM for 72 h. Cells were collected and stained with an Annexin V PE apoptosis detection kit (BD Biosciences) to determine the percentage of apoptotic cells. Immunoblotting and binding assay To detect CD11b expression on B cells, highly purified FO B cells or MZ B cells were sorted from CD11b WT or KO mice. For B cell signalling studies, purified B cells (4 × 10 6 ) were stimulated with anti-IgM (40 μg ml −1 ) at 37 °C for the indicated time points. Cells were subsequently lysed in Triton X-100 lysis buffer containing protease and phosphatase inhibitors. The whole-cell extracts were separated by SDS–polyacrylamide gel electrophoresis and electrotransferred to polyvinylidene difluoride membrane. After blocking, the membranes were probed overnight at 4 °C with appropriate primary Abs (1:1000 or 1:2000 dilution) and then secondary Ab (1:3000 dilution). The blots were developed using ECL Plus Western Blotting Detection Reagents (GE Healthcare). For CD22 immunoprecipitation, purified B cells (2.5 × 10 7 ) or transfected B cell line (1.5 × 10 7 ) were left unstimulated or with anti-IgM and lysed in 1% NP-40 lysis buffer containing protease inhibitor and phosphatase inhibitor. The lysates were precleared with protein A/G plus-agarose (Santa Cruz Biotechnology) by rotation for 1 h at 4 °C, and then incubated with anti-CD22 (Southern Biotech, clone 2D6) overnight at 4 °C. Immune complexes were isolated by adsorption to protein A/G plus-agarose for additional 4 h at 4 °C. Beads were washed two times with lysis buffer with no NP-40 and boiled in sample buffer for 5 min. The samples were separated by SDS–polyacrylamide gel electrophoresis and then immunoblotted with antibodies against total phosphotyrosine, SHP-1, Lyn, FLAG and CD22. All full blots are displayed in Supplementary Fig. S6 . To measure the binding of CD22 to CD11b, CD11bWT- and CD11b Mut-transfected CHO-K1 cells were incubated with recombinant human CD22 his tag protein (10 μg ml −1 ) for 60 min at 4 °C followed by mouse anti-His tag and fluorescein isothiocyanate (FITC)-labelled anti-mouse IgG monoclonal Abs. Cells were analysed by flow cytometry. In some experiment, CD11bWT-transfected CHO-K1 cells were pretreated with neuraminidase (Sigma) for 3 h and then used for CD22-binding assay. Quantitative real-time PCR B cells from WT and CD11b KO anti-snRNP Ig Tg mice were stimulated with or without anti-IgM (40 μg ml −1 ). RNAs were extracted with Trizol (Life Technologies). After reverse transcription into complementary DNA with a Reverse Transcription Kit (Bio-Rad), quantitative PCR was then performed on Bio-Rad MyiQ single colour RT–PCR detection system using SYBR Green Supermix. Gene-specific primers are summarized in the Supplementary Table S1 . We normalized gene expression level to β-2 microglobulin (β-MG) housekeeping gene and represented data as fold differences by the 2 −ΔΔCt method, where ΔCt=Ct target gene −Ct β-MG and ΔΔCt=ΔCt induced −ΔCt reference . Calcium influx assays Calcium mobilization was monitored in Indo-1-loaded cells stimulated with anti-IgM. Purified B cells or transfected B cell lines were resuspended at 2 × 10 6 ml −1 , loaded with 1.5 μl pluronic acid (Ana Spec Inc) and 2 μl Indo-1 (Life Technologies) for 30 min at 37 °C. After incubation, the cells were washed and resuspended in Ca 2+ -free Hank’s balanced salt solution. Calcium traces were recorded in a HITACHI fluorescence spectrometer with an excitation wavelength of 355 nm and an emission wavelength of 405 nm. After the establishment of a stable baseline, the cells were stimulated with anti-IgM, followed by the addition of CaCl 2 at a final concentration of 1 mM. In vivo BrdU incorporation assay B10.A CD11b WT or KO anti-snRNP Ig Tg mice received 1 mg BrdU in 0.1 ml PBS via intraperitoneal injection at day 1 and 0.8 mg ml −1 BrdU in their drinking water between days 1 and 5. BrdU staining was performed and analysed using flow cytometry. In vivo immunization and autoAb detection Age-matched B10.A CD11b WT or KO anti-snRNP Ig Tg mice were immunized by intravenous injection of 2 × 10 7 apoptotic thymocytes weekly for 9 weeks. The sera were collected at indicated time points. Detection of anti-snRNP by enzyme-linked immunosorbent assay (ELISA) was done using recombinant snRNP D protein as a coating Ag on ELISA plates. ANA was detected by indirect immunofluorescence. Serum samples were diluted 1:10 in PBS and placed onto HEp-2 cell-coated slides (Antibodies Incorporated) and incubated for 1 h in a humidified container. Each slide was washed with PBS before addition of FITC-conjugated anti-mouse IgG (eBiosciences) and humid incubation for an additional 1 h. To detect kidney Ig deposition, cryostat frozen sections were fixed in ice-cold acetone and blocked with BSA in PBS. IgG deposition was detected with HRP (horseradish peroxidase)-conjugated sheep anti-mouse IgG (1:25, Amersham). Slides were developed with 3-amino-9-ethylcarbazole substrate solution (Vector Laboratories). Images were obtained using Nikon ECLIPSE Ti fluorescence microscopy or acquired by Aperio ScanScope digital scanner. B cell transfer in Rag1 - and B cell-deficient μMT mice Splenic B cells and CD4 + T cells from C57Bl/6 CD11b WT or KO anti-snRNP Ig Tg mice were enriched by magnetic bead-positive selection and depletion using anti-CD4 microbeads and anti-CD43 microbeads (Miltenyi Biotech). B (15 × 10 6 ) and T cells (5 × 10 6 ) were injected intravenously into Rag1- deficient mice. Five days after cell transfer, recipients were immunized with apoptotic thymocytes for six times. For B cell-deficient μMT mouse adoptive transfer experiment, CD11b WT or KO B cells (15 × 10 6 ) were adoptively transferred into μMT mice. Mice were immunized with apoptotic thymocytes for four times and anti-snRNP autoAb was detected by ELISA. BM transplantation Mice were lethally irradiated with 950 cGy from a γ-irradiation source. After 16 h, mice were transplanted with 1 × 10 7 BM cells from B10.A CD11b WT or KO anti-snRNP Ig Tg mice. The B cell development and function were assessed 28 days after transplantation. Generation of stable CD11b-expressing B cell lines Human CD11b was amplified from CD11b plasmid (plasmid 8631, Addgene) with primers listed in the Supplementary Table S1 . PCR product was cloned into plasmid c-Flag pcDNA3 (plasmid 20011, Addgene). This plasmid contains a single carboxy-terminal Flag-tag sequence. To generate site-directed mutation of CD11b, the QuikChange II XL Site-directed mutagenesis kit (Stratagene) was used. Constructs were verified by sequencing. K46-17 cells and α2,6-sialyltransferase-positive CHO-K1 cells from Dr. Vaclav Vetvicka of University of Louisville were transfected with plasmid using MicroPulser electroporator (Bio-Rad). After 24 h, transfected cells were selected in medium containing G418. CD11b-expressing K46-17 cells and CHO-K1 cells were purified by two rounds of sorting and cloning by limiting dilution. Expression of CD11b was analysed using flow cytometry and western blot. Co-localization analysis Cells were left unstimulated on ice or stimulated for 10–30 min at 37 °C with biotin-labelled anti-IgM. Cells were fixed and permeabilized using Perm/Wash buffer and then incubated with streptavidin-phycoerythrin and antibodies against CD11b, CD22, SHP-1 and phospho-Lyn (Y396) in Perm/Wash buffer. The samples were acquired using Amnis ImageStream system (Amnis Corporation) and analysed using IDEAS analysis software (Amnis Corporation). The degree of co-localization was analysed using similarity feature. Detection of sialic acids Expression of sialic acids on WT or R77H-mutated CD11b was detected by lectin binding [33] using flow cytometry. Briefly, WT or R77H-mutated CD11b-transfected CHO-K1 cells were incubated with biotinylated lectin S. nigra (Vector Laboratories) at 10 μg ml −1 for 60 min on ice. Cells were washed twice and then stained with streptavidin-FITC. Parental CHO-K1 cells were used as controls. Expression of sialic acids was detected by flow cytometry. Statistical analysis Data are expressed as means±s.e.m. Statistical significance of difference was determined by the unpaired two-tailed Student’s t -test. Differences were considered significant for P <0.05. Statistical analysis was performed using Prism 4.0 (GraphPad Software). How to cite this article: Ding, C. et al . Integrin CD11b negatively regulates BCR signalling to maintain autoreactive B cell tolerance. Nat. Commun. 4:2813 doi: 10.1038/ncomms3813 (2013).